Rates of speciation and morphological evolution are correlated across the largest vertebrate radiation Several evolutionary theories predict that rates of morphological change should be positively associated with the rate at which new species arise. For example, the theory of punctuated equilibrium proposes that phenotypic change typically occurs in rapid bursts associated with speciation events. However, recent phylogenetic studies have found little evidence linking these processes in nature. Here we demonstrate that rates of species diversification are highly correlated with the rate of body size evolution across the 30,000+ living species of ray-finned fishes that comprise the majority of vertebrate biological diversity. This coupling is a general feature of fish evolution and transcends vast differences in ecology and body-plan organization. Our results may reflect a widespread speciational mode of character change in living fishes. Alternatively, these findings are consistent with the hypothesis that phenotypic ‘evolvability’—the capacity of organisms to evolve—shapes the dynamics of speciation through time at the largest phylogenetic scales. The striking differences in both species richness and morphological diversity that exist between major groups of organisms constitute a ubiquitous yet unexplained pattern in the large-scale organization of biological diversity. Some groups, such as African cichlids, have rapidly diversified into a vast number of species and functional forms. This exceptional diversity contrasts with the many groups that contain few species and/or harbour comparatively little phenotypic or ecological diversity. As first recognized by Darwin, some groups—lungfishes, coelacanths and others—are virtual ‘living fossils’ and have been characterized by low species diversity and morphological stasis for much of their evolutionary history [1] . Paleontologists have long suspected that these observations reflect a fundamental coupling between rates of cladogenic speciation and morphological evolution [1] , [2] . Many studies have tested whether concerted shifts in speciation (cladogenesis) and morphological evolution occur through time during adaptive radiation or after mass extinction within single groups [3] , [4] , [5] , [6] . However, we know little about the extent to which these rates are coupled across multiple contemporaneous lineages and the effect of this coupling on standing patterns of biological diversity. The theory of punctuated equilibrium proposed that morphological change typically occurs in association with speciation events [7] , [8] , but palaeontological tests of the model have typically focused on patterns of morphological change associated with particular speciation events [9] , [10] or general patterns of morphological stasis through time [11] . These studies have not tested whether per-lineage rates of phenotypic evolution are correlated with per-lineage rates of cladogenic speciation. Most research on the causes of evolutionary rate variation among extant groups has considered species diversification and phenotypic evolution in isolation, and the few studies that have directly addressed the coupling of these rates have obtained negative [12] or conflicting results [13] , [14] . Here we examine the relationship between rates of cladogenic speciation and rates of body size evolution across ray-finned fishes (Actinopterygii), a major evolutionary radiation that includes approximately half of all known species of vertebrates. We generated a time-calibrated phylogeny for 7,822 extant fish species that span the entire spectrum of actinopterygiian diversity. As no methods are available for explicitly modelling the relationship between rates of species diversification and rates of phenotypic evolution, we developed a Bayesian framework for jointly estimating these parameters as well as their evolutionary correlation across the branches of phylogenetic trees. We used this phylogenetic data set and methodological framework to test whether the processes of species diversification and morphological evolution were coupled during the radiation of living fishes. Phylogenetics and diversification modelling We assembled a time-calibrated phylogeny for living fishes (Methods and Supplementary Methods ) using a mega-phylogeny approach [15] . Our phylogenetic tree included representatives of nearly all species with DNA sequence data available in public sequence repositories and was temporally calibrated with 60 fossils ( Supplementary Data 1 and Supplementary Tables S1 and S2 ). We assembled body size data for 6,760 species from Fishbase, the most comprehensive source of biological data on the world’s fishes [16] . We developed a novel methodological framework to study the evolutionary correlation between rates of speciation and phenotypic evolution (see Methods and Supplementary Methods ). Our approach does not rely on any a priori classification of lineages into particular clades or named higher taxa (for example, ‘Cichlidae’), but assumes that the phylogeny and associated phenotypic data were generated under a heterogeneous mixture of evolutionary rates. The model (BAMM; Bayesian Analysis of Macroevolutionary Mixtures) uses reversible-jump Markov Chain Monte Carlo to automatically detect subtrees that share common evolutionary parameters of speciation, extinction and body size evolution ( Fig. 1 ). Rates were allowed to shift along any of the 15,647 branches in the fish tree, and rate shifts (‘events’) were added to and removed from the tree under a compound Poisson process [17] . Our approach is related to recent reversible-jump Markov Chain Monte Carlo methods for studying trait evolution in isolation [12] , [18] but jointly accounts for speciation, extinction and the correlation between these parameters and rates of trait evolution. Our tree contains ~27% of known fish species and the level of sampling varies considerably among fish families ( Fig. 2 ). As incomplete taxon sampling can lead to biased estimates of speciation and extinction on molecular phylogenies [19] , [20] , we analytically accounted for missing species in our likelihood calculations using clade-specific sampling fractions ( Fig. 2 and Supplementary Methods ). 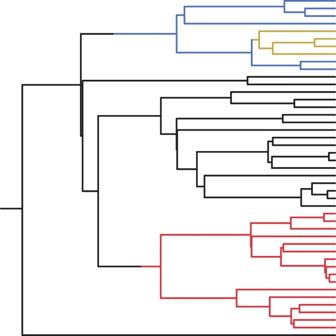Figure 1: Multiple evolutionary processes on a phylogenetic tree. The hypothetical tree is painted with a collection of four processes (black, gold, blue and red), each of which reflects a distinct set of macroevolutionary (speciation, extinction, and trait evolution) parameters. Black represents the processΦRassociated with the root node; all descendant lineages inheritΦRuntil reaching a tip or untilΦRis terminated by a ‘downstream’ event. Events can occur at any position along a branch, and a single branch can thus be subdivided into sections belonging to different events. In addition, subtrees defined by events can be rendered paraphyletic by the occurrence of new events on sublineages. In this example, this occurs for both the root process (rendered paraphyletic by the occurrence of blue, red and gold processes), as well as the blue process (rendered paraphyletic by the gold process). Figure 1: Multiple evolutionary processes on a phylogenetic tree. The hypothetical tree is painted with a collection of four processes (black, gold, blue and red), each of which reflects a distinct set of macroevolutionary (speciation, extinction, and trait evolution) parameters. Black represents the process Φ R associated with the root node; all descendant lineages inherit Φ R until reaching a tip or until Φ R is terminated by a ‘downstream’ event. Events can occur at any position along a branch, and a single branch can thus be subdivided into sections belonging to different events. In addition, subtrees defined by events can be rendered paraphyletic by the occurrence of new events on sublineages. In this example, this occurs for both the root process (rendered paraphyletic by the occurrence of blue, red and gold processes), as well as the blue process (rendered paraphyletic by the gold process). 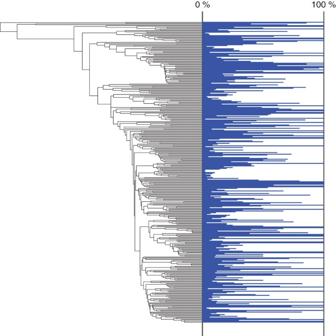Figure 2: Degree of incomplete taxon sampling varies by family. Shown (blue) is the percentage of recognized species diversity within each fish family that was included in the full 7,822 taxon fish tree. These clade-specific sampling probabilities were used to correct for incomplete taxon sampling in the BAMM analyses. Full size image Figure 2: Degree of incomplete taxon sampling varies by family. Shown (blue) is the percentage of recognized species diversity within each fish family that was included in the full 7,822 taxon fish tree. These clade-specific sampling probabilities were used to correct for incomplete taxon sampling in the BAMM analyses. Full size image Our results overwhelmingly support multiple evolutionary rate shifts across the time-calibrated fish tree. The mean of the posterior distribution of log-likelihoods from a simple model with a single rate of speciation, extinction and trait evolution (three parameters) was −37,842 (0.025 and 0.975 quantiles of −38,022 and −37,654, respectively). Allowing rate-shift events to pop on and off of the tree under a compound Poisson process resulted in a massive improvement to the log-likelihood of the data ( Supplementary Fig. S1 ); the mean of the posterior density of log-likelihoods for the full model was −32,694 (0.025 and 0.975 quantiles of −32,904 and −32,492, respectively). The median of the posterior distribution of the number of rate shifts was 65 (0.025 and 0.975 quantiles of 62 and 69, respectively; Supplementary Fig. S2a ). The mean rate of speciation across the entire evolutionary history of fishes ( N =7,822) was 0.141 lineages per million years (my), and the mean rate of extinction was 0.043 lineages per my. Our mean estimate of the ratio of extinction to speciation was 0.284 ( Supplementary Fig. S2b ); this is perhaps lower than expected based on the fossil record, but far higher than the near-zero results frequently reported in phylogenetic studies. Relationship between speciation and body size evolution Our results indicate a striking positive relationship between the rate of speciation and the rate of log-transformed body size evolution ( Fig. 3 ). This pattern is not driven by one or several clades, but appears to be a general feature of fish evolution: both rapidly and slowly evolving clades are distributed widely across the 7,864 taxon fish tree ( Fig. 3a ). The mean phylogenetically independent correlation ( Fig. 3b and Supplementary Methods ) between log-transformed rates of speciation and phenotypic evolution across the full tree was 0.642 ( P <0.001); rank correlations were nearly identical ( r =0.654, P <0.001). 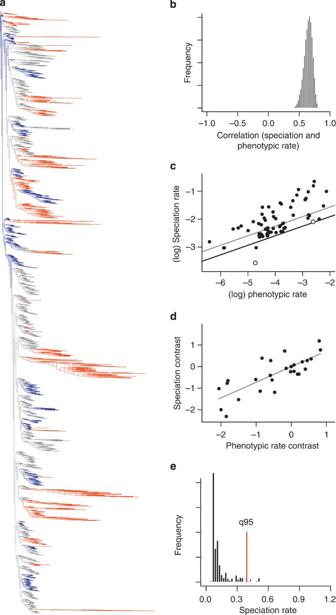Figure 3: Rates of speciation and body size evolution across ray-finned fishes. (a) Full tree of 7,824 taxa showing evolutionary rates from BAMM analysis. Branch lengths are proportional to estimated speciation rates; red/blue branches denote rates of body-size evolution that fall into the upper and lower quartiles of branch rates. Rates on red branches are at least 2.5-fold greater than those on the fastest blue branches. (b) Posterior distribution of the correlation between log-transformed rates of speciation and phenotypic evolution. (c) Mean log-transformed speciation rates and phenotypic rates for all fish families with at least five sampled species. PGLS regressions are computed for teleost families (n=170; black circles; grey line) and for all fishes (black line; open circles denote the two non-teleost clades). (d) Contrasts between speciation rates and phenotypic rates for sister clades only (n=48). (e) Distribution of speciation rates across all 7,822 species of fish included in the analysis. Red line (q95) denotes the 0.95 quantile of the distribution of rates; maximum observed rate was 1.27 lineages per my. Regression slopes incanddare highly significant (P<10−10). Figure 3: Rates of speciation and body size evolution across ray-finned fishes. ( a ) Full tree of 7,824 taxa showing evolutionary rates from BAMM analysis. Branch lengths are proportional to estimated speciation rates; red/blue branches denote rates of body-size evolution that fall into the upper and lower quartiles of branch rates. Rates on red branches are at least 2.5-fold greater than those on the fastest blue branches. ( b ) Posterior distribution of the correlation between log-transformed rates of speciation and phenotypic evolution. ( c ) Mean log-transformed speciation rates and phenotypic rates for all fish families with at least five sampled species. PGLS regressions are computed for teleost families ( n =170; black circles; grey line) and for all fishes (black line; open circles denote the two non-teleost clades). ( d ) Contrasts between speciation rates and phenotypic rates for sister clades only ( n =48). ( e ) Distribution of speciation rates across all 7,822 species of fish included in the analysis. Red line (q95) denotes the 0.95 quantile of the distribution of rates; maximum observed rate was 1.27 lineages per my. Regression slopes in c and d are highly significant ( P <10 −10 ). Full size image We computed mean rates of speciation and body size evolution across branches for each recognized family of fish that was represented by at least five species in the full tree. Phylogenetic generalized least squares (PGLS) regression indicates a highly significant positive relationship between these parameters ( Fig. 3c , black line; PGLS slope=0.60; P <10 −15 , df=172; all rates log-transformed for regression analyses). PGLS intercepts are highly sensitive to the leveraging effect of early diverging and species-poor lineages; when we removed the two non-teleost lineages from the analysis (sturgeons and gars), we recovered an identical slope but different intercept ( Fig. 3c , grey line; PGLS slope=0.60; P <10 −15 ; df=170). Virtually identical results were obtained using regressions of independent contrasts through the origin ( Supplementary Fig. S3 ). Thus, our central result cannot be explained by the presence of early diverging, species-poor lineages and does not depend on the choice of analytical method. As an additional check on our results, we collapsed the full fish tree to family-level clades and found maximum likelihood estimates of rates of speciation and trait evolution under several evolutionary models without BAMM. Analysis of these family-specific rate estimates using PGLS indicate a highly significant correlation between net speciation rate and the rate of body size evolution under several background extinction regimes ( Fig. 4a ; P <0.002). 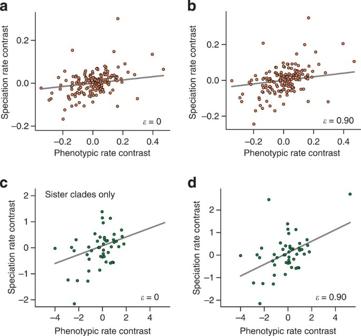Figure 4: Maximum likelihood analyses of relationship between rates of body-size evolution and speciation. (a,b) Relationship between speciation rate and rate of log-transformed body size evolution, using maximum likelihood estimates of rates for 163 fish families. Shown are phylogenetic independent contrasts between the logarithm of the speciation rate and the logarithm of the rate of phenotypic evolution under two relative extinction rates (= 0.90 corresponds to an extinction rate equal to 90% of the speciation rate). (c,d) Relationship between contrasts in log-transformed phenotypic evolutionary rates and log-transformed speciation rates for sister clades only (n= 49 pairs of clades) under two relative extinction rates. All analyses indicate that these rates are positively correlated (P= 0.002; df = 1, 47). Spearman's rank correlation between these contrasts is also significant= 0: r = 0.30,P= 0.035;= 0.90:r= 0.35,P= 0.013). As contrasts are restricted to clades of identical age, this relationship is unlikely to result from the confounding effects of age on estimates of either speciation rates or rates of body size evolution. Figure 4: Maximum likelihood analyses of relationship between rates of body-size evolution and speciation. ( a , b ) Relationship between speciation rate and rate of log-transformed body size evolution, using maximum likelihood estimates of rates for 163 fish families. Shown are phylogenetic independent contrasts between the logarithm of the speciation rate and the logarithm of the rate of phenotypic evolution under two relative extinction rates ( = 0.90 corresponds to an extinction rate equal to 90% of the speciation rate). ( c , d ) Relationship between contrasts in log-transformed phenotypic evolutionary rates and log-transformed speciation rates for sister clades only ( n = 49 pairs of clades) under two relative extinction rates. All analyses indicate that these rates are positively correlated ( P = 0.002; df = 1, 47). Spearman's rank correlation between these contrasts is also significant = 0: r = 0.30, P = 0.035; = 0.90: r = 0.35, P = 0.013). As contrasts are restricted to clades of identical age, this relationship is unlikely to result from the confounding effects of age on estimates of either speciation rates or rates of body size evolution. Full size image Sister clade contrasts and time scaling of rates The analysis of correlations between evolutionary rates can be confounded if diversification rates within clades have slowed through time and if morphological space is saturated [21] . To address this, we compared contrasts in evolutionary rates for sister clades only. By focusing exclusively on contrasts between sister clades, we thus compare rates only between clades of identical age, thereby eliminating potentially spurious correlations attributable to age variation alone. Even after restricting our analysis to sister clades only, we find a significant relationship between maximum likelihood estimates of the rate of speciation and the rate of phenotypic evolution ( Fig. 4c ). Under both relative extinction scenarios, contrasts in (log-transformed) rates of phenotypic evolution predict contrasts in (log-transformed) rates of speciation ( Fig. 4c ; P <0.001; df=1, 47). The Spearman’s rank correlation between these contrasts is also significant ( ε =0: r =0.30, P =0.035; ε =0.90: r =0.35, P =0.013). Together, these results indicate that the correlation between speciation and the rate of body size evolution is unlikely to result from a confounding effect of clade age alone. When we computed mean evolutionary rates for families using branch-specific BAMM estimates, we likewise observed a significant positive correlation ( Fig. 3d ; r =0.75; P <10 −10 ; df=1, 62). The number of sister clades for the maximum likelihood analyses ( N =49) differed from the total for the BAMM analyses ( N =63), because maximum likelihood estimates required that we exclude clades where taxon sampling was insufficient to capture the crown age of the clade with high probability (Methods and Supplementary Methods ). Although speciation and extinction rates are correlated across the tree ( ρ =0.83; P <0.001), we found no evidence that the relative extinction rate—the ratio of extinction to speciation—is related to rates of phenotypic evolution. Neither the relative extinction rate, nor its interaction with speciation, was a significant predictor of phenotypic evolutionary rates (PGLS: P >0.45; df=172), although speciation remained highly significant with these terms in the PGLS regression model ( P <10 −10 ). It is unlikely that an indirect correlation with extinction drives the patterns we report here for extant lineages, although selective extinction has clearly been important across the history of fishes [22] . Speciation rate variation across living fishes Rapidly diversifying groups of animals tend to dominate published summaries of speciation rate variation [23] , [24] , in part because of research bias towards such clades. Our analyses provide a first glimpse at the frequency distribution of speciation rates in the natural world at the level of individual lineages ( Fig. 3e ) that is largely independent of researcher bias. Although some lineages are characterized by exceptionally high speciation rates, many lineages in the fish phylogeny show minor deviations from the global average rate: more than 50% of all sampled fish lineages ( N =4,848) are estimated to have speciation rates that lie between 0.078 and 0.14 lineages per my. To assess clade-specific variation in rates of species diversification and body size evolution, we computed mean evolutionary rates for each family from branch-specific estimates ( Fig. 5 ). Cichlids rank near the top in both the rate of speciation and rate of body size evolution. Salmonids also fall into the fastest decile for both evolutionary rates. This pattern may be largely driven by the explosive diversification of Coregonus whitefishes and Salvelinus chars in postglacial North American and Eurasian lakes, consistent with previous research demonstrating that members of this group can rapidly diversify into distinct morphologies in response to ecological niche availability [25] , [26] , [27] . Sebastidae represents another exceptionally fast clade, potentially reflecting recent adaptive radiation in temperate Pacific rockfishes [28] , [29] . 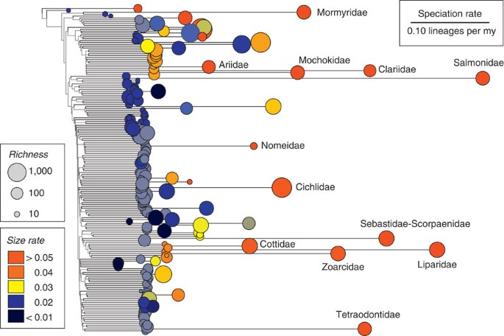Figure 5: Mean speciation and phenotypic evolutionary rates across a family-level tree of living fishes. Terminal branch lengths are proportional to speciation rates; tip size and colours represent extant species richness and rate of body size evolution. Labelled clades denote families that fall in the fastest 10% for both the rate of speciation and the rate of phenotypic evolution. Tree includes all families represented by five or more species (n=172) in the full tree. Figure 5: Mean speciation and phenotypic evolutionary rates across a family-level tree of living fishes. Terminal branch lengths are proportional to speciation rates; tip size and colours represent extant species richness and rate of body size evolution. Labelled clades denote families that fall in the fastest 10% for both the rate of speciation and the rate of phenotypic evolution. Tree includes all families represented by five or more species ( n =172) in the full tree. Full size image However, a number of clades that are not traditionally recognized as ‘exceptional’ fall into the fastest decile of rates ( Fig. 5 ). These include the African electric fishes (Mormyridae), snailfishes (Liparidae), driftfishes (Nomeidae), eelpouts (Zoarcidae), sculpins (Cottidae) and three families of African freshwater catfishes (Ariidae, Mochokidae and Clariidae). The slowest decile of rates for both speciation and phenotypic evolution includes several families whose extant members are highly similar to fossil forms. These include the bonytongues (Osteoglossidae) and gars (Lepisosteidae), the latter being the very first group referenced by Darwin when he introduced the phrase ‘living fossil’ to the lexicon of evolutionary biology [30] . The correlation between speciation and phenotypic evolution has left a clear signal on the extant biota that can be recovered from molecular phylogenies of living species alone, a result that contrasts sharply with recent studies, suggesting a decoupling of these processes [12] . Contrasts between high-rate and low-rate lineages appear to be a pervasive feature of fish evolution ( Fig. 3a ), and our results imply that this correlation has influenced nearly half of vertebrate diversity. The patterns we report here could result, in part, from at least two potential sampling phenomena. The first involves the well-documented ‘time scaling’ of evolutionary rates, such that older lineages appear to undergo slower morphological change (or species diversification) relative to younger lineages [14] , [31] , [32] . A number of potential explanations have been advanced for this phenomenon, both real and artefactual [14] , [32] , [33] . These problems are particularly acute when using ‘constant-rate’ diversification models. In the case of speciation, diversity-dependent slowdowns in the rate of cladogenesis through time can lead to apparent time-scaling of rates, such that constant-rate estimates of speciation will be negatively correlated with clade age [34] , [35] . A similar phenomenon can occur for morphological evolutionary rates if morphospaces become saturated through time [36] , [37] . Saturation of ‘species space’ and ‘morphological space’ can thus result in negative correlations between evolutionary rates and time, and potentially (and indirectly) generate artefactual correlations between speciation rates and morphological rates. Our sister clade analyses ( Fig. 4c ), by restricting inference to contrasts between clades of identical age, indicates that such time scaling alone is unlikely to explain our results. A second sampling phenomenon is more insidious and involves biases resulting from taxonomic practice. If taxonomists are more likely to split morphologically variable lineages into multiple species, then we might have observed higher speciation rates in those same lineages that show exceptional morphological diversity. At present, we can simply acknowledge that such biases may exist and have the potential to impact all macroevolutionary analyses at this scale. Ideally, all species units would be delimited using an identical and quantitative set of criteria [38] , but we are far from achieving this in practice. More importantly, it is not clear which direction such taxonomic biases should go: it is also possible that taxonomists are less likely to recognize lineages that show considerable morphological variation. For example, many species of fish in postglacial lakes show substantial polymorphism with reproductive isolation (for example, whitefishes, chars and sticklebacks) [25] , [27] , yet owing to the recency of divergence between these partially or fully isolated lineages they are not recognized as distinct species. This bias would be conservative with respect to the findings of our study. We considered only a single axis of phenotypic variation—body size—and we predict that similar results will follow from considering the evolution of multidimensional phenotypes. An interesting exception to our general results involves sturgeons (Acipenseridae), an early-diverging fish lineage that has long been considered a ‘living fossil’ [1] , [39] . Although fossil sturgeons are exceedingly similar to extant sturgeons in overall form, the group shows considerable variation in body size, from Pseudoscaphirhynchus dwarf sturgeons to Huso huso , one of the largest living actinopterygiians. Our analyses identify sturgeons as having one of the fastest overall rates of body size evolution, roughly 5.4-fold higher than the median rate across all lineages. Despite these elevated rates of body size evolution, we predict that sturgeons will be characterized by low rates of body shape evolution relative to many other fish lineages. These results suggest that two of the most widely celebrated features of extant fish diversity—living fossils and adaptive radiations—reflect endpoints of an evolutionary trend that has played out over hundreds of millions of years. This connection between speciation and morphological evolution is partly consistent with traditional formulations of punctuated equilibrium [7] , whereby the speciation process itself leads to morphological change. However, an alternative explanation for this result is that phenotypic evolvability—the capacity of lineages to evolve morphological and ecological novelty—itself promotes speciation [40] , [41] . Many biologists already recognize this notion intuitively as the mechanism by which ecological key innovations promote diversification during adaptive radiation [42] , [43] , [44] . Unlike punctuated equilibrium, a coupling between evolvability and speciation provides an immediate explanation for the observation that speciation rates themselves vary widely among clades ( Figs 3 , 4 , 5 ), as well as the phylogenetic predictability of adaptive radiation [45] , [46] . We are only beginning to understand the developmental genetic and ecological mechanisms that might underlie clade-specific differences in evolvability [40] , but some evidence suggests that clades vary substantially in their capacity to evolve novel phenotypes [43] , [47] , [48] . At present, we are unable to distinguish between punctuated equilibrium and evolvability-diversification correlations as mechanisms underlying the observed positive relationship between rates of speciation and of phenotypic evolutionary rates [49] . Nonetheless, our analysis suggests that the differential proliferation of morphologically fast and slow lineages has profoundly influenced the diversity of living fishes. Matrix assembly and phylogenetic methods We identified a set of 13 genes with high coverage across fishes (see Supplementary Methods ) and assembled gene region matrices using the Phylogeny Assembly with Databases tool ( http://phlawd.net [15] ). All profile sequence alignments were conducted using MUSCLE (v. 3.6; [50] ) and standard sequence alignments were conducted with MAFFT (v. 6.86 (ref 51 )). We used the FishBase systematic classification to organize data acquisitions, to identify synonymies and to map common names to species. Within a set of synonyms, we assembled chimeric sequences to maximize coverage within and across our 13-gene data set. We concatenated all 13 alignments to produce a final matrix with 13 gene regions and 7,822 taxa for phylogenetic analysis (86.13% missing data across 11,621 sites). We inferred a maximum likelihood topology using RAxML 7.2.8 (refs 52 , 53 ), assuming a number of topological constraints to increase computational efficiency, minimize the influence of rogue taxa on topology [54] , [55] and maximize taxon sampling ( Supplementary Methods ). We assumed γ-distributed rate heterogeneity (GTRGAMMA) and implemented the rapid hill-climbing algorithm introduced by Stamatakis [52] . We used joint branch-length optimization across 13 (gene) partitions. Penalized likelihood dating analyses [56] were conducted using the treePL programme ( http://github.com/blackrim/treepl ). This programme allows for better optimization with enormous trees by combining stochastic optimization with hill-climbing gradient-based methods. As rates were assumed to be extremely non-clock-like, a low smoothing value of 1e−5 was chosen. The rate-smoothed phylogeny was deposited in Dryad ( doi:10.5061/dryad.j4802 ). Bayesian analysis of macroevolutionary mixtures We modelled the evolution of diversification rates across the fish tree by assuming that the phylogeny was shaped by a mixture of evolutionary processes of speciation, extinction and trait evolution. The model proposes that ‘events’, or rate shifts, are added to or removed from the phylogeny according to a compound Poisson process [17] . The occurrence of an event on a particular branch v e defines an ‘event subtree’ τ e : all nodes and branches descended from v e inherit the collection of evolutionary processes Φ 1 (defined by the event at v e ), until the event is terminated. An event terminates at terminal branches or at the next downstream event ( Fig. 1 ). Each event and associated subtree τ e was associated with three parameters: a speciation rate ( λ ), an extinction rate ( μ ), and a rate of phenotypic evolution ( β ). In the analyses presented here, we assumed that rates of speciation, extinction and trait evolution were constant across all regions of the phylogeny defined by a particular event ( Fig. 1 ); and also that these rates were constant in time. The rate of trait evolution was simply the evolutionary rate under a Brownian motion process of trait evolution, such that the variance in the expected value of a given phenotypic state after some amount of time t was given by βt . The occurrence of an event thus induces decoupling between the parent rates and all downstream evolutionary rates. To compute the likelihood of a phylogeny with character state data at the tips, we assumed independence of the character states and diversification rates, such that the joint likelihood of the data was given by L ( τ , ω )= L ( τ ) L ( ω ), where τ is the tree and ω is a vector of phenotypic data. We computed the likelihood of each event subtree τ e under the corresponding constant-rate birth-death process ( Supplementary Methods ). We analytically accounted for missing taxa in our likelihood calculations ( Supplementary Methods ). Although our sampling included 27% of total actinopterygiian diversity, this percentage varied considerably among clades ( Fig. 2 ). We modified our likelihood equations to incorporate family-specific sampling fractions, to account for this sampling heterogeneity across clades. Our model explicitly allows extinction rates to exceed speciation rates for any given event subtree. We implemented the model in a Bayesian framework, integrating over prior distributions to obtain marginal distributions of evolutionary rates for each branch in the fish tree. Under a compound Poisson process, the number of events on the tree is a Poisson-distributed random variable that occurs with rate Λ . These events can change position, can be deleted from the tree and occur on any branch with a probability proportional to the length of the branch. There is no upper bound on the number of events, as multiple events can occur on each branch. The full model contains the following parameters: the overall event rate Λ ; the root rates λ R , μ R and β R ; λ , μ and β , and location parameters for each event; and ancestral character states for each internal node in the tree. We used the Metropolis–Hastings–Green algorithm [57] to construct a Markov chain that allowed movement between model spaces of different dimensionality, as occurs when events are added to or deleted from the tree. When an event was added to the tree, all branches and nodes downstream of the new event ‘belong’ to the event, and they are governed by the evolutionary rates (for example, Φ 1 =( λ 1 , μ 1 , β 1 )) associated with the event. Following the addition of an event to the tree, the evolutionary rates are set equal to those of the preceding event. The addition of a new event on some subtree would result in a new collection of processes or rates ( Φ 1 ). Initially, these new rates are set to be equal to the parent rates, but they are decoupled and can rapidly diverge. Likewise, deletion of an event collapses rates on all branches governed by a given event to the rates associated with the parent event. In the preceding example, deletion of the single event would involve setting all branches/nodes governed by Φ 1 to the parent process at the root ( Φ R ). A tree with 0 events is governed strictly by the evolutionary processes at the root and would only contain three parameters in the current model formulation ( λ R , μ R , β R ). There is no upper bound on the number of events, as multiple events can occur on each branch. The Jacobian for transdimensional moves (additions and deletions) is 1 (ref. 17 ); all proposal ratios have been derived previously [17] and are described in detail in the Supplementary Methods . To directly estimate the evolutionary correlation between the rate of speciation and rate of phenotypic evolution, we simply consider that each collection of processes Φ on the fish phylogeny are independent from rates on any other parts of the tree, because a rate-shift event by definition decouples these rates from other regions of the tree. The evolutionary correlation between rates can thus be computed simply from the collection of processes Φ x ( x 1, 2,...., N ), where there are N such processes on the tree. We performed a set of simulations to verify that our implementation of the model did not result in artefactual correlations between speciation and trait evolution when no such relationship existed ( Supplementary Methods and Supplementary Fig. S4b ). Maximum likelihood analyses We tested the relationship between rates of log-transformed body size evolution and speciation rates using a conventional maximum likelihood framework, estimating rates of speciation and phenotypic evolution for each fish family independently. We used phylogenetic independent contrasts to analyse the phylogenetic correlation between log-transformed rates. We computed the maximum likelihood estimate of the rate of phenotypic evolution for each clade under Brownian motion [58] , [59] . We then estimated the net diversification rate for each group using crown-clade estimators [60] under several relative extinction rates ( ε =0; ε =0.90) given the observed clade diversity, then back-computed the speciation rate for the clade from these values. As taxon sampling was incomplete, we only estimated rates for clades where our phylogeny had a probability of 0.80 or greater of containing the true root node for each family ( Supplementary Methods ). Perhaps the most serious artefact that could confound our analyses of the correlation between speciation and the rate of phenotypic evolution would occur if both rates are confounded with time [14] . For example, it is well known that constant-rate estimators of diversification rates can covary with clade age if clade diversity is limited by ecological factors [35] . To address this possibility, we performed a second set of contrast-based analyses, but restricted our analysis to sister clades. We thus considered only clades of equal age. If the pattern we report here is driven solely by the confounding effect of time on evolutionary rate estimates, then we should not observe a significant relationship using sister clade contrasts. ‘Old’ sister clades may have low rates for both speciation and phenotypic evolution and ‘young’ sister clades may have fast rates, but there is no reason to predict a coupling between these rates if the pattern is strictly an artefact of clade age. How to cite this article: Rabosky, D. L. et al. Rates of speciation and morphological evolution are correlated across the largest vertebrate radiation. Nat. Commun. 4:1958 doi: 10.1038/ncomms2958 (2013).